Imprintable membranes from incomplete chiral coalescence Coalescence is an essential phenomenon that governs the equilibrium behaviour in a variety of systems from intercellular transport to planetary formation. In this report, we study coalescence pathways of circularly shaped two-dimensional colloidal membranes, which are one rod-length-thick liquid-like monolayers of aligned rods. The chirality of the constituent rods leads to three atypical coalescence pathways that are not found in other simple or complex fluids. In particular, we characterize two pathways that do not proceed to completion but instead produce partially joined membranes connected by line defects— π -wall defects or alternating arrays of twisted bridges and pores. We elucidate the structure and energetics of these defects and ascribe their stability to a geometrical frustration inherently present in chiral colloidal membranes. Furthermore, we induce the coalescence process with optical forces, leading to a robust on-demand method for imprinting networks of channels and pores into colloidal membranes. Driven by surface tension, a pair of liquid droplets undergo a large-scale transformation as they merge into a single daughter droplet. In order for the droplets to coalesce, a rupture must occur between two merging interfaces which, coupled with surface tension and hydrodynamic forces, leads to energetic barriers and non-trivial coalescence progression [1] , [2] , [3] , [4] , [5] . For complex fluids with partial positional and/or orientational order, the complexity of the coalescence reactions increases considerably [6] . A well-studied example belonging to this category is lipid vesicles, whose fusion is characterized by complex barriers that include structural distortions, which expose the hydrophobic core of the lipid bilayer and allow the merger to proceed [7] , [8] , [9] . In addition to fluid droplets and vesicles, coalescence is also important in the formation of solid structures such as carbon nanotubes or sintered powders [10] , [11] . In most cases, coalescence is an ‘all-or-none’ process; once initiated, the reaction proceeds to completion. However, moving along a complex-free energy landscape, there is also the possibility of a coalescence reaction that overcomes an initial energy barrier only to get trapped in an intermediate state, such as merging vesicles producing a hemi-fused state or coalescing nanotubes producing a defect-ridden structure [10] , [12] . Here we study the coalescence pathways of two-dimensional (2D) colloidal membranes composed of liquid monolayers of aligned rod-like viruses [13] . We present coalescence dynamics markedly different from that observed between either simple liquid droplets or complex lipid vesicles. The chirality of the constituent rod-like viruses introduces an insurmountable topological barrier that suppresses the conventional coalescence pathway observed between liquid droplets and greatly slows down the coarsening dynamics. Instead, the coalescence proceeds by atypical higher-order pathways to intermediate states in which two membranes are joined together by 1D defects. The topology of these intermediate structures suppresses the subsequent kinetic step, resulting in the robust formation of two types of line defects whose stability is only limited by the sample lifetime. Theoretical work and computer simulations predict that colloidal membranes are an equilibrium phase that should be observed in diverse suspensions of highly anisotropic monodisperse rods with attractive interactions [14] , [15] . In the same way that disclination lines are intimately connected and influence the properties of nematic liquid crystals, the defects described here are a ubiquitous feature of colloidal membranes. The colloidal nature of our building blocks allows us to characterize the structure and dynamics of membrane-imprinted defects in great detail using several complementary microscopy techniques. This enables us to formulate and quantitatively test a theoretical model of π -walls. Furthermore, we engineer coalescence events using optical forces in order to create well-defined networks of 1D channels or pores embedded within a 2D colloidal membrane. Using such technology, we imprint and analyse excitations with skyrmion topology, an important class of defects that has recently been studied in varied soft and hard materials [16] , [17] , [18] , [19] , [20] , [21] . Three coalescence pathways We use fd wild-type ( wt) viruses, which are rod-like colloidal particles with 880 nm contour length, 7 nm diameter and 2.8 μm persistence length [22] . Adding non-adsorbing polymer induces effective attractive interactions between otherwise electrostatically repulsive rods through the well-studied depletion mechanism [23] . Under specific conditions, the depleting agent condenses homogeneous rod-like viruses into colloidal membranes, one rod-length-thick chiral smectic-A (Sm- A *) monolayers of aligned rods whose continuum properties are identical to those of conventional lipid bilayers [13] , [14] . A feature that critically affects the coalescence pathways is the membrane's edge, consisting of a twisted layer of rods that penetrate a small distance into the membrane interior ( Fig. 1a,b ) [24] , [25] . Rod tilting is enforced by surface tension, which is minimized for a curved edge. The chirality of fd wt rods is left handed [26] , [27] , which imposes a well-defined handedness onto the colloidal membrane edge. This complex edge behaviour is one specific manifestation of a very general packing frustration present whenever chiral molecules are forced to assemble into 2D smectic-like sheets [28] , [29] , [30] , [31] . 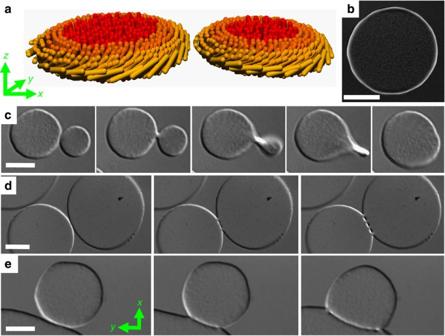Figure 1: Three coalescence pathways of colloidal membranes. (a) Colloidal membranes in which surface tension induces tilting of the rods at the edge. 180° of twist is trapped at the proximal edges of the membranes. (b) A 2D-LC-PolScope image of a colloidal membrane, in which the intensity at each pixel is proportional to the magnitude of the local retardance. The bright ring along the membrane periphery indicates local rod tilting. (c) A coalescence pathway resulting in a defect-free daughter membrane. The coalescing membranes initially form a twisted bridge that induces a torque onto the smaller membrane, rotating it by 180° and expelling the twist (Supplementary Movie 1). (d) A coalescence pathway resulting in the formation of an alternating bridge-pore array (Supplementary Movie 2). (e) A coalescence pathway resulting in the formation of aπ-wall. The membranes have sedimented onto the coverglass surface that, for sufficiently massive membranes, suppresses the rotation required for defect-free coalescence (Supplementary Movie 3). Scale bars, 10 μm. Figure 1: Three coalescence pathways of colloidal membranes. ( a ) Colloidal membranes in which surface tension induces tilting of the rods at the edge. 180° of twist is trapped at the proximal edges of the membranes. ( b ) A 2D-LC-PolScope image of a colloidal membrane, in which the intensity at each pixel is proportional to the magnitude of the local retardance. The bright ring along the membrane periphery indicates local rod tilting. ( c ) A coalescence pathway resulting in a defect-free daughter membrane. The coalescing membranes initially form a twisted bridge that induces a torque onto the smaller membrane, rotating it by 180° and expelling the twist ( Supplementary Movie 1 ). ( d ) A coalescence pathway resulting in the formation of an alternating bridge-pore array ( Supplementary Movie 2 ). ( e ) A coalescence pathway resulting in the formation of a π -wall. The membranes have sedimented onto the coverglass surface that, for sufficiently massive membranes, suppresses the rotation required for defect-free coalescence ( Supplementary Movie 3 ). Scale bars, 10 μm. Full size image In contrast to lipid bilayers that assemble into edgeless three-dimensional (3D) vesicles, colloidal monolayer membranes appear as flat 2D disks with exposed edges. As two co-planar membranes approach laterally, chirality causes the rods at the proximal membrane edges to be tilted in opposite directions, trapping 180° of twist between them ( Fig. 1a ). After a coalescence event, these rods end up in the membrane interior where they are forced to untwist by the global assembly constraints. The energetic cost associated with a pathway in which the peripheral rods untwist and two co-planar membranes coalesce laterally is prohibitively large and is never observed. Rather, we have identified three alternate types of coalescence events that proceed along more complex pathways. This unique behaviour arises specifically due to the chiral topological barrier imposed by the 180° of twist trapped between the two merging edges. The first pathway results in the formation of defect-free daughter membranes and shares certain similarities as well as important differences with the well-studied coalescence of liquid droplets ( Fig. 1c , Supplementary Movie 1 ). Similar to liquid droplets, thermally induced fluctuations cause the merging membranes to rupture and establish a one rod-length-thick bridge between them. Within such a bridge, rods twist by 180° in order to match the orientations of the joining edges. The over-twisted bridge induces a torque that rotates the two membranes in order to expel the trapped twist. As the membranes twist around each other, the connecting bridge expands in width, eventually producing a circularly shaped defect-free daughter membrane. In conventional coalescence, the rate of neck expansion is determined by hydrodynamic and inertial forces [3] . By contrast, the significantly slower neck expansion in membrane coalescence is dominated by the rate at which the two membranes rotate with respect to each other. In the second pathway, coalescing membranes simultaneously rupture at multiple locations, forming many collinear twisted bridges separated by depletant-filled pores ( Fig. 1d , Supplementary Movie 2 ). These bridges eventually multiply and spread along the periphery of the coalescing structures, resulting in membranes that are joined through a 1D array of pores that alternate with one-rod-length-thick twisted bridges (alternating bridge-pore arrays, ABPAs). The third coalescence pathway ( Fig. 1e , Supplementary Movie 3 ) is initiated by establishing two twisted necks, which hold the membranes together and induce the nucleation of a continuous 1D line defect. This uniform defect, called a π -wall because it traps 180° of twist, quickly grows to its equilibrium size, pushing the two necks apart. Once a π -wall or ABPA is formed, the topological barrier for a subsequent transition to a lower energy defect-free membrane involves untwisting of defect-bound rods and cannot be overcome on experimental timescales. Coalescence on demand Molecular chirality introduces frustration into the coalescence of colloidal membranes, resulting in the formation of 1D defects ( Fig. 1 ). However, being a consequence of random coalescence events, the spatial location of such defects is impossible to control. It is therefore desirable to develop a robust on-demand method for imprinting defects into colloidal membranes with arbitrary spatial precision, similar to recent work with thermotropic liquid crystals [32] , [33] , [34] . We demonstrate that membrane self-coalescence can be induced with optical forces ( Fig. 2 ), opening up the possibility of engineering well-defined 2D defect networks. Moving an optical trap from a membrane's edge into the interior results in the creation of two edges aligned along the direction of trap translation ( Fig. 2a ). Subsequently, a π -wall nucleates between these two edges and grows in length, zipping up the gap created by the translating optical trap. If the trap is released in the membrane interior, the π -wall quickly retracts ( Supplementary Movie 4 ). However, moving the trap to the distal edge anchors the π -wall, making it stable indefinitely. This method makes it possible to imprint a complex, predesigned interconnected network of π -walls into a large membrane ( Supplementary Movie 5 ). Such networks can serve as templates for the assembly of colloidal particles, which are stably trapped for indefinitely long periods of time at the junction of three π -walls ( Supplementary Fig. 1 ) [17] . The same technique is used to imprint an ABPA as well as transform a π -wall into an ABPA and vice versa ( Fig. 2b , Supplementary Movies 6 and 7 ). These results demonstrate that the unique coalescence of fd membranes coupled with accessibility of colloidal systems to direct manipulation leads to assembly of tunable membrane landscapes. 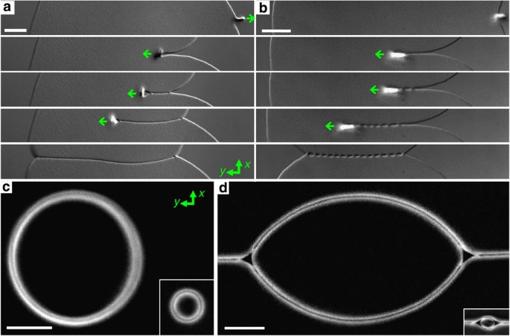Figure 2: Imprinting defects with optical forces. (a) An optical trap moving from the edge of a membrane towards the interior initiates the formation of aπ-wall by artificially creating a coalescence event (Supplementary Movie 5). Translating the trap across the entire membrane results in the formation of a stableπ-wall. Green arrows indicate the trap translation direction. (b) Under conditions where ABPAs are favored, creating a coalescence event results in the formation of a stable ABPA. (c) Complex structures imprinted into membranes using optical forces. A 2D-LC-PolScope image of aπ-wall ring. (d) A 2D-LC-PolScope image of twoπ-wall triple junctions. Over time these structures shrink to their equilibrium sizes shown in the insets and determined by the balance of line tension and bending rigidity. Scale bars, 10 μm (a,b), 5 μm (c,d, including insets). Figure 2: Imprinting defects with optical forces. ( a ) An optical trap moving from the edge of a membrane towards the interior initiates the formation of a π -wall by artificially creating a coalescence event ( Supplementary Movie 5 ). Translating the trap across the entire membrane results in the formation of a stable π -wall. Green arrows indicate the trap translation direction. ( b ) Under conditions where ABPAs are favored, creating a coalescence event results in the formation of a stable ABPA. ( c ) Complex structures imprinted into membranes using optical forces. A 2D-LC-PolScope image of a π -wall ring. ( d ) A 2D-LC-PolScope image of two π -wall triple junctions. Over time these structures shrink to their equilibrium sizes shown in the insets and determined by the balance of line tension and bending rigidity. Scale bars, 10 μm ( a , b ), 5 μm ( c , d , including insets). Full size image Structure of π -wall and pore defects To characterize π -wall defects, we prepared samples containing a low fraction of fluorescently labelled viruses, allowing us to track dynamics of individual particles ( Fig. 3a,b , Supplementary Movie 8 ). For membranes lying in the image ( x - y ) plane, fluorescently labelled rods in the membrane interior, aligned along the z -axis, appear as isotropic spots. In the vicinity of a π -wall, particles become elongated, indicating local twisting. To confirm the proposed structure, we use 2D-LC-PolScope microscopy, a technique that produces images in which each pixel's intensity is proportional to the 2D projection of the sample optical retardance, R (ref. 35 ). There is no structural or optical anisotropy in the membrane interior, hence this region appears black when viewed with LC-PolScope ( Fig. 3c ). Tilting of rods away from the monolayer normal melts the smectic order into a nematic (cholesteric) ( Fig. 3g ), resulting in structural and optical anisotropy in the x - y plane that becomes visible as a bright birefringent band with LC-PolScope. Thus, the bright region observed along the length of the π -wall supports the hypothesis that rods twist by 180° across the defect. Furthermore, 3D-LC-PolScope reveals that rods within the π -wall have left-handed twist, in agreement with measurements in the bulk cholesteric phase ( Fig. 3e,f , Methods) [22] , [36] . 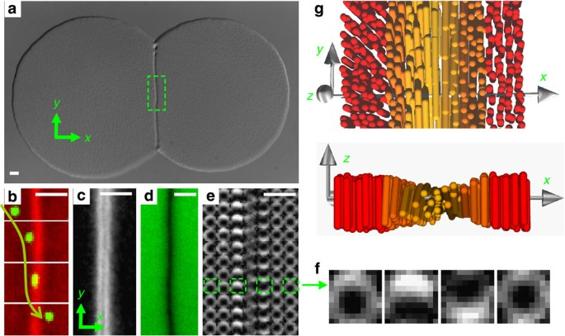Figure 3: Complimentary microscopy techniques reveal the structure of aπ-wall. (a) A differential interference microscopy image of aπ-wall embedded in a colloidal membrane. (b) A time sequence illustrates rotation of a fluorescently labelled virus (green) by 180° as it diffuses through aπ-wall (Supplementary Movie 8). Fluorescence images are overlayed with simultaneously acquired phase-contrast images (red). (c) A 2D-LC-PolScope image of aπ-wall. The magnitude of the local retardance is mapped onto a linear grey scale that ranges fromR=0 nm (black) toR=4 nm (white). (d) A fluorescence image of aπ-wall in which all the rods are fluorescently labelled. The defect appears darker than the membrane bulk, indicating a local decrease in membrane thickness. (e) A 3D-LC-PolScope image determines the 3D orientation of the viruses across aπ-wall. (f) The four dotted green boxes in (e), illustrating the shift of the dark zero-retardance spot in 3D-LC-PolScope along a transverse cut through the defect (see Methods). (g) Schematic illustration of aπ-wall. Scale bars, 2 μm. Figure 3: Complimentary microscopy techniques reveal the structure of a π -wall. ( a ) A differential interference microscopy image of a π -wall embedded in a colloidal membrane. ( b ) A time sequence illustrates rotation of a fluorescently labelled virus (green) by 180° as it diffuses through a π -wall ( Supplementary Movie 8 ). Fluorescence images are overlayed with simultaneously acquired phase-contrast images (red). ( c ) A 2D-LC-PolScope image of a π -wall. The magnitude of the local retardance is mapped onto a linear grey scale that ranges from R =0 nm (black) to R =4 nm (white). ( d ) A fluorescence image of a π -wall in which all the rods are fluorescently labelled. The defect appears darker than the membrane bulk, indicating a local decrease in membrane thickness. ( e ) A 3D-LC-PolScope image determines the 3D orientation of the viruses across a π -wall. ( f ) The four dotted green boxes in ( e ), illustrating the shift of the dark zero-retardance spot in 3D-LC-PolScope along a transverse cut through the defect (see Methods). ( g ) Schematic illustration of a π -wall. Scale bars, 2 μm. Full size image Using the same microscopic techniques, we also elucidate the structure of ABPAs ( Fig. 4a ). 2D-LC-PolScope reveals twisting of rods within the smectic bridges ( Fig. 4b ), and this is confirmed by tracking individual fluorescently labelled rods ( Fig. 4c ). Images of membranes assembled from 100% fluorescently labelled rods indicate local membrane density. In such images, pores appear dark indicating that they are filled with the depleting polymer ( Fig. 4d ). A schematic of a bridge-pore array is shown in Fig. 4e . 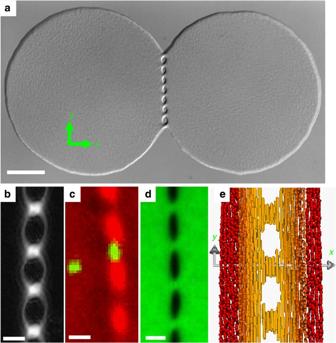Figure 4: An ABPA embedded in a colloidal membrane. (a) A differential interference microscopy image of an alternating array of pores and twisted smectic bridges (ABPA) joining two membranes. (b) A 2D-LC-PolScope retardance image indicates rod twisting within the bridges. (c) Simultaneous fluorescence (green) and phase-contrast (red) imaging reveals rod twist within a smectic bridge. (d) An ABPA in which all the rods are fluorescently labeled reveals that the pores are empty of virus particles. (e) A schematic diagram of an ABPA. Scale bars, 10 μm (a) and 2 μm (b–d). Figure 4: An ABPA embedded in a colloidal membrane. ( a ) A differential interference microscopy image of an alternating array of pores and twisted smectic bridges (ABPA) joining two membranes. ( b ) A 2D-LC-PolScope retardance image indicates rod twisting within the bridges. ( c ) Simultaneous fluorescence (green) and phase-contrast (red) imaging reveals rod twist within a smectic bridge. ( d ) An ABPA in which all the rods are fluorescently labeled reveals that the pores are empty of virus particles. ( e ) A schematic diagram of an ABPA. Scale bars, 10 μm ( a ) and 2 μm ( b – d ). Full size image Theoretical model of the π -wall When viewed with 2D-LC-PolScope, the centre of a π -wall appears darker as evidenced by a local minimum in the intensity profile ( Fig. 5a ). 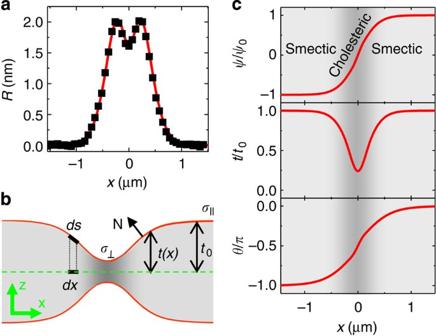Figure 5: Theoretical model quantitatively describes theπ-wall structure. (a) A retardance profile taken along a transverse cut through aπ-wall defect exhibits two peaks. Experimental data (black squares) is quantitatively described by the theoretical model (red curve). The centre of theπ-wall lies atx=0. (b) A schematic of a transverse cut through aπ-wall. Dark grey shaded area indicates the region where tilting of the rods locally melts the smectic into a cholesteric, while the light grey shaded area indicates the Sm-A* region.t0is the thickness of the bulk membrane andt(x) is the local thickness. The surface normalis in the (x,z)-plane.σ|andσ⊥indicate the bulk membrane surface tension and theπ-wall surface tension, respectively. (c) Plots of the variation of the smectic order parameter normalized by its bulk value (Ψ/Ψ0), the thickness profile (t/t0) and the tilt angle (θ/π) across aπ-wall. To understand this, we note that the retardance of a colloidal membrane lying in the image plane is given by: Figure 5: Theoretical model quantitatively describes the π -wall structure. ( a ) A retardance profile taken along a transverse cut through a π -wall defect exhibits two peaks. Experimental data (black squares) is quantitatively described by the theoretical model (red curve). The centre of the π -wall lies at x =0. ( b ) A schematic of a transverse cut through a π -wall. Dark grey shaded area indicates the region where tilting of the rods locally melts the smectic into a cholesteric, while the light grey shaded area indicates the Sm- A * region. t 0 is the thickness of the bulk membrane and t ( x ) is the local thickness. The surface normal is in the ( x , z )-plane. σ | and σ ⊥ indicate the bulk membrane surface tension and the π -wall surface tension, respectively. ( c ) Plots of the variation of the smectic order parameter normalized by its bulk value (Ψ/Ψ 0 ), the thickness profile ( t / t 0 ) and the tilt angle ( θ / π ) across a π -wall. Full size image where n =4.1 × 10 −5 ml mg −1 is the specific birefringence of a fully aligned bulk sample at unit concentration [37] , t is the membrane thickness, S is the nematic order parameter (assumed equal to 1), c is the local concentration of virus and θ is the tilt angle of rods away from the layer normal ( z -axis) [25] . Since the retardance increases with increasing θ , a π -wall with unchanging thickness would yield a singly peaked function. A profile with two peaks separated by a local minimum indicates reduced membrane thickness at the π -wall centre ( Fig. 5a ). To disentangle the contribution of varying θ and t to the overall retardance profile, we develop a theoretical model of a π -wall. We model the π -wall by a Ch region sandwiched between two semi-infinite Sm- A * monolayers. Our model utilizes the de Gennes free energy density f Ch-A for the Ch-Sm- A * transition (Methods) [38] , [39] , [40] , [41] . The free energy per unit length of a Sm- A * flat layer in the x - y plane containing a π -wall is given by: The volume terms in square brackets are multiplied by the local thickness t ( x ). The smectic order parameter Ψ describes the transition from a Sm- A * monolayer of aligned rods to a Ch region. The only contribution to f Ch−A from the Frank free energy density is the twist term, as the nematic director n rotates by an angle θ about the x -axis within a characteristic length scale λ t , the twist penetration depth [25] . The second term dictates that t = t 0 (see Fig. 5b ) in the bulk region of fully aligned fd viruses (Ψ=Ψ 0 ), and that t is decoupled from the orientation of n in the cholesteric region (Ψ=0). v is the Lagrange multiplier due to the volume constraint of the membrane. The constants in the fourth and fifth terms of equation (2) are the bulk surface tension modulus σ | when n | , and the π -wall surface tension modulus σ ⊥ when n ⊥ , where is the local unit normal of the curved membrane surface ( Fig. 5b ). ds is the infinitesimal arc length of the surface, and its projection onto the x -axis is dx ( Fig. 5b ). In the presence of anisotropy ( σ | ≠ σ ⊥ ), the local surface tension changes continuously due to the local tilt of n between the two regimes. The last term in equation (2) is the free energy cost of the surface curvature [42] . The π -wall thickness profile is determined by the competition between surface and volume contributions to the free energy. Since tilting of the rods raises free energy, the volume term favors thinner π -wall profiles. The surface term associated with the rod–polymer interface favors a thicker π -wall profile with uniform thickness that minimizes the exposed surface. The mean-field analysis of equation (2) predicts how the membrane thickness t , virus tilt angle θ and smectic order parameter Ψ vary across a π -wall ( Fig. 5c ). The variation of Ψ demonstrates the continuous melting of the Sm- A * into a Ch phase at the centre of a π -wall. This data, along with theoretical predictions for θ and t in equation (1), yield a retardance profile that fits the experimental data and determines the twist penetration depth, λ t ( Fig. 5a , Supplementary Table 1 ). A best fit to experimental results is achieved for a membrane thickness at the π -wall centre of 220 nm, significantly smaller than the 880 nm thickness of the membrane interior. Thus, π -walls form deep channels within a monolayer of otherwise uniform height. This finding can be directly confirmed by fluorescence microscopy where the image intensity is directly proportional to local membrane thickness; a π -wall is significantly darker than the membrane bulk ( Fig. 3d ). π -wall energetics and stability π -wall defects exhibit significant fluctuations that are observable with optical microscopy ( Fig. 6a , Supplementary Movie 9 ). The analysis of such fluctuations yields a spectrum from which it is possible to extract the π -wall line tension, γ π and bending rigidity, κ π (Methods, Fig. 6b ) [24] , [43] . We determine the dependence of γ π and κ π on relevant molecular parameters, namely fd chirality and depletant osmotic pressure ( Fig. 6c ). Chirality is tuned by temperature; at T =60 °C, the rods are achiral (no twisting) and chirality increases with decreasing temperature [24] . Stronger chiral interactions result in larger twist angles required to minimize the rod interaction energy. Virus concentration within a membrane is determined by the osmotic pressure of the surrounding depletant and increases with increasing Dextran concentration. For comparison, we have also analysed fluctuations of an exposed membrane edge to extract its line tension ( γ edge ) and bending rigidity ( κ edge ) [24] . 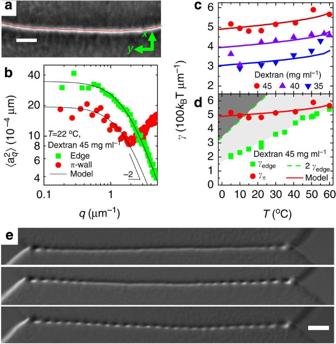Figure 6: Fluctuations reveal the line tensionγπand bending rigidityκπof aπ-wall. (a) A phase-contrast image of aπ-wall (Supplementary Movie 9). Scale bar, 2 μm. (b) A fluctuation spectrum of the membrane's edge (green squares) and aπ-wall (red circles) as a function of the wave vectorq. The data are fitted with=kBT/(γ+κq2). (c) Dependence ofγπ(solid markers) on sample temperature (fdchirality) for three different Dextran concentrations.γπis fitted with the theoretical model (equation (2)). (d) Comparison ofγπandγedgeas a function of temperature for a dextran concentration of 45 mg ml−1. The dashed green line indicates 2γedge. As a first approximation, we expect that forγedge<γπ<2γedge(light grey shading),π-walls are stable with respect to two free membrane edges, whereas forγπ>2γedge(dark grey shading),π-walls are metastable with respect to unbound membranes. (e) A temperature quench induces a transition from aπ-wall into an ABPA. The colloidal membrane assembled at 45 mg ml−1Dextran is quenched fromT=55 to 22 °C. During the quench, the two membranes joined by aπ-wall locally dissociate by the formation of pores. However, instead of complete dissociation the two membranes remain joined by the array of smectic bridges. The pores nucleate at the edges and propagate towards the middle of theπ-wall (Supplementary Movie 10). The transition is reversible, and with increasing temperature, an ABPA transforms back into aπ-wall. Scale bar, 5 μm. Figure 6: Fluctuations reveal the line tension γ π and bending rigidity κ π of a π -wall. ( a ) A phase-contrast image of a π -wall ( Supplementary Movie 9 ). Scale bar, 2 μm. ( b ) A fluctuation spectrum of the membrane's edge (green squares) and a π -wall (red circles) as a function of the wave vector q . The data are fitted with = k B T /( γ + κq 2 ). ( c ) Dependence of γ π (solid markers) on sample temperature ( fd chirality) for three different Dextran concentrations. γ π is fitted with the theoretical model (equation (2)). ( d ) Comparison of γ π and γ edge as a function of temperature for a dextran concentration of 45 mg ml −1 . The dashed green line indicates 2 γ edge . As a first approximation, we expect that for γ edge < γ π <2 γ edge (light grey shading), π -walls are stable with respect to two free membrane edges, whereas for γ π >2 γ edge (dark grey shading), π -walls are metastable with respect to unbound membranes. ( e ) A temperature quench induces a transition from a π -wall into an ABPA. The colloidal membrane assembled at 45 mg ml −1 Dextran is quenched from T =55 to 22 °C. During the quench, the two membranes joined by a π -wall locally dissociate by the formation of pores. However, instead of complete dissociation the two membranes remain joined by the array of smectic bridges. The pores nucleate at the edges and propagate towards the middle of the π -wall ( Supplementary Movie 10 ). The transition is reversible, and with increasing temperature, an ABPA transforms back into a π -wall. Scale bar, 5 μm. Full size image For a wide range of parameters, we find that κ π is consistently equal to 2 κ edge and is independent of the physical parameters, which is reasonable since the twist penetration region of a π -wall is twice that of an exposed edge [24] . We obtain values of κ π and κ edge of about 200 k B T μm and 100 k B T μm, respectively, and these values do not change significantly with varying polymer concentration or rod chirality. By contrast, γ π and γ edge exhibit more complex dependence on microscopic parameters. Strengthening chirality raises the free energy of untwisted rods in the interior while lowering the free energy of twisted edge- or defect-bound rods, thus lowering γ (ref. 24 ). We find that π -walls are always metastable with respect to the untwisted bulk phase ( γ π >0) but that chirality can reduce γ π by up to 100 k B T μm −1 . Increasing rod attraction (increasing dextran concentration) significantly raises γ π , and this increase does not depend on molecular chirality ( Fig. 6c ). Our theoretical model predicts γ π = F − F bulk , where F bulk and F are the free energy per unit length of a monolayer of perfectly aligned rods and a π -wall, respectively (equation (2)). Fitting chirality-dependent γ π ( Fig. 6d ) and the retardance profiles ( Fig. 5a ), and using the previously measured value of K 2 (ref. 26 ), we determine the parameters in equation (2): λ t , k , σ | and σ ⊥ ( Supplementary Table 1 ). k , σ | and σ ⊥ are determined by the polymer concentration and are independent of chirality, in agreement with experiments. The retardance profiles are independent of both chirality and polymer concentration ( Supplementary Fig. 2 ). As a first approximation, when γ edge becomes larger than γ π , we might expect a spontaneous dissociation of a π -wall into two defect-free membranes. We search for such an event by performing a temperature quench of a π -wall, which quickly increases the strength of chirality. Surprisingly, instead of dissociation, we observe a transition of π -walls into ABPAs ( Fig. 6e , Supplementary Movie 10 ). Pores nucleate from the ends of the π -wall and propagate into the interior of the line defect. The π -wall-to-ABPA transition is reversible; with increasing temperature, an ABPA transforms back into a π -wall. ABPAs are more frequently observed in the high chirality limit, while π -walls tend to be more stable for weakly chiral rods. This behaviour is reasonable, as pores create a large amount of rod–polymer interface that is favored at higher chirality [24] . For many parameters we observe coexisting ABPAs and π -walls ( Supplementary Fig. 1 ) indicating a substantial kinetic barrier associated with transformation between these structures. Engineering complex defect structures With detailed understanding of the dynamics, structure and energetics of π -walls, we are in a position to engineer defects that are inaccessible through natural coalescence processes. As an example, we have used optical tweezers to sever a π -wall in two places, and then quickly joined the two ends to form a closed ring within the membrane interior ( Fig. 2c ). These particle-like structures are similar to skyrmion excitations in that they have positive energy compared with the background field, but remain indefinitely stable as there is an insurmountable barrier to their excision from the host membrane [18] , [19] , [20] . The equilibrium size of a π -wall ring is determined by the competition between two effects: the interfacial energy, F i =2 πγ π r , and the bending energy, F b =2 πκ π / r , where r is the radius of the ring. The first term favors smaller rings, while the second term favors structures with larger radius and lower curvature energy. Once created, a π -wall ring slowly shrinks, ultimately reaching an equilibrium radius of r eq =1.3 μm at T =22 °C (inset Fig. 2c , Supplementary Fig. 3 ). Minimizing the free energy that contains both line tension and bending rigidity terms predicts that r eq = . We can also estimate from the corner spatial frequency of the fluctuation spectrum ( Fig. 6b ). For the same parameters, the π -wall fluctuation spectrum yields r eq = =0.65 μm. The discrepancy between these two methods is likely due to the high curvature of skyrmion-like defects, requiring an expansion of the bending energy to higher orders than 1/ r 2 . Besides skyrmions, it is also possible to imprint other shapes such as triple junctions, for which a similar analysis can be performed ( Fig. 2d , Supplementary Fig. 4 , Methods). Taken together, these examples illustrate the potential of the imprinting technique to investigate the universal behaviour of various topological defects embedded in 2D membranes. We have described three coalescence pathways of chiral colloidal membranes. Two pathways do not proceed to completion but instead remain stuck indefinitely in a local energy minimum, producing membranes that are partially joined by 1D line defects that trap chiral twist. We have formulated a comprehensive theoretical model of chiral π -wall defects and quantitatively tested it against extensive experimental data. Numerous theoretical works, computer simulations and experiments have demonstrated that fd viruses used in our studies are an excellent experimental realization of hard rods [22] , an important model system that has been studied for many decades. It follows that the phenomenology we describe should be relevant to diverse colloidal and nanosized rods that interact through excluded volume interactions. From an application perspective, aligned monolayers of semiconducting rods have diverse applications ranging from light emitting diodes to photovoltaic devices [44] , and colloidal membranes offer an easily scalable method for assembling such structures. Understanding the principles that promote or inhibit membrane coarsening and defect formation described here is essential for obtaining large-scale monodomain samples. Our work demonstrates that rod chirality inhibits membrane coalescence and coarsening, thus suppressing formation of macroscopic membranes. Consequently, it also suggests that engineering colloidal membranes from achiral rod-like subunits would lead to formation of defect-free uniform monolayers. Sample preparation Bacteriophage fd viruses were grown in the XL1-Blue E. Coli. strain and purified as described previously [24] . Optical microscopy chambers were assembled using glass slides and cover slips (Goldseal, Fisher Scientific) with an unstretched parafilm layer acting as a spacer as discussed previously [24] . Optical microscopy methods Experiments were carried out on an inverted microscope (Nikon TE-2000) equipped with traditional polarization optics, a differential interference contrast (DIC) module, a fluorescence imaging module and a 2D-LC-Polscope module [45] . We used a 100 × oil immersion objective (PlanFluor NA 1.3 for DIC and PlanApo NA 1.4 for phase contrast). Images were recorded with cooled CCD cameras (CoolSnap HQ (Photometrics, Tuscon, AZ) or Retiga Exi (QImaging, Surrey BC, Canada)). For 3D-LC-PolScope measurements, we used a Zeiss Axiovert 200 M microscope with a Plan Apochromat oil immersion objective (63X/1.4NA), and a monochrome CCD camera (Retiga 4000 R, QImaging, Surrey BC, Canada) [35] . Temperature was regulated in situ with a Peltier device equipped with a proportional integral derivative temperature controller (ILX Lightwave LPT 5910). The temperature controlling side of the Peltier is attached to a copper ring fitted to the size of the microscope objective. A thermistor, placed in the copper ring adjacent to the sample, permits the proportional integral derivative feedback necessary to adjust the temperature. The excess heat is removed with constant flow of room temperature water on the other side of the Peltier device. Using this setup, we control the temperature anywhere between 4 and 60 °C. Fluctuations of the π -wall and membrane edges were analysed using previously described methods [24] , [46] . For analysis of π -wall fluctuations, we used phase-contrast microscopy instead of DIC. This ensured that the intensity profile along transverse cuts through the defect contour would be Gaussian-shaped, which is optimal for tracking. The lower performance of phase-contrast imaging results in a larger signal-to-noise for the π -wall spectra when compared with the analysis of the membrane edge acquired with DIC imaging. The 2D-LC-PolScope cannot distinguish between clockwise and counterclockwise rod tilting. To determine the twisting direction, we utilized the 3D-LC-PolScope ( Fig. 3e,f ), which yields a full 3D retardance map of the membrane [24] , [45] . A microlens array, introduced into the image plane of the objective lens, produces a grid of conoscopic microimages on the CCD camera, with each microimage determining the local rod orientation. An azimuthally symmetric retardance profile with a centred dark spot indicates that rods are locally oriented along the z -axis, as observed in the membrane interior ( Fig. 3e ). A shift of the dark zero-retardance spot away from the centre of a conoscopic image indicates the magnitude of the local tilting of the rods, while its azimuthal angle indicates the direction of the birefringence vector projection in the x - y plane ( Fig. 3e ). Using 3D-LC-PolScope, we demonstrate that the π -walls embedded in fd membranes have left-handed twist, similar to the handedness of the bulk cholesteric phase [22] , [36] . Optical tweezers Colloidal membranes were manipulated with a holographic optical tweezer setup built around an inverted Nikon TE-2000 microscope. A 1,064 nm laser beam (Compass 1064, Coherent) is expanded by a telescope and reflected at near-normal incidence off of a liquid-crystal-on-silicon spatial light modulator (SLM) (Hamamatsu, X10468-03). The SLM is imaged onto the back focal plane of the objective lens using a second telescope, which also shrinks the beam to slightly overfill the back aperture of the objective lens. The phase mask encoding the hologram is calculated and displayed on the SLM using a modified version of freely available software [47] . Using this software, multiple point traps were created and translated in the image plane in real time. Complements on the π -wall theory We assume that membranes and π -walls formed by filamentous fd viruses are type-II smectic materials, based on the analogy with superconductors [40] , [41] . In other words, the coherence length ξ , the length scale of the relaxation of the smectic order, is much smaller than the twist penetration depth λ t , confirmed by the agreement of previous theories based on the Frank free energy of monolayers with experiments [13] , [39] , [48] . Moreover, we assume a linear π -wall, so that the fields in equation (2) depend only on x . The de Gennes free energy density [40] , [41] for the cholesteric-Sm- A * transition due to distortions of the nematic director n ≡{0,sin θ ( x ),cos θ ( x )} in a semi-infinite membrane, f Ch−A , in equation (2) is given by [13] , [39] Ψ is the real part of the complex order parameter , and the first three terms in equation (3) describe the crossover from a one rod-length-thick monolayer of perfectly aligned fd (Ψ=Ψ 0 = ) to the cholesteric region forming around the π wall (Ψ=0). The change in the phase of due to big distortions of n and arising from t ≠cos θ near the π -wall is absorbed in the fourth term of equation (3) and in the second term of equation (2) without loss of generality, ensuring rotational invariance. The length scales are given by λ t ≡ and ξ i ≡ . Using the boundary conditions that θ =0, Ψ=Ψ 0 , t = t 0 , as well as their vanishing derivatives of every order in the bulk monolayer, θ = , Ψ=0, t = and =0 at the midline of the π-wall, the thickness t , tilt angle θ and smectic order parameter Ψ are numerically calculated by solving Euler–Lagrange equations minimizing equation (2). π -wall and membrane edge fluctuation analysis To measure γ π , we determine the instantaneous π -wall configuration with sub-pixel precision [46] . The conformation of the interface, described by the local tangent angle α ( y ) at position y along the line defect, is decomposed into a Fourier series: α ( y )= a q sin( qy ). Analysing a series of uncorrelated images yields the fluctuation spectrum (mean square Fourier amplitudes versus wave vector q ). There are two contributions to the free energy of a fluctuating π -wall defect F fluct : a line tension term proportional to the overall defect length, and an elastic energy term proportional to the local defect curvature. The origin of the curvature term is the melting of the smectic monolayer into a nematic in the vicinity of the π -wall defect. It follows that the free energy of a fluctuating π -wall is given by: F fluct leads to the fluctuation spectrum = k B T /( γ + κq 2 ), and fitting this expression to the experimentally measured curve yields values for γ π and κ π ( Fig. 6b ). Repeating the same analysis for the exposed membrane edge yields its line tension ( γ edge ) and bending rigidity ( κ edge ) as discussed previously [24] ( Fig. 6b ). The contrast of π -wall images is significantly lower when compared with those of an exposed edge, resulting in a π -wall fluctuation spectrum that is dominated by noise for q >2 μm −1 . In comparison, the fluctuation spectrum of an exposed edge extends to much higher q values. Complements on π -wall triple junction structure π -wall triple junction structures are created from a single π -wall by forming a second π -wall connecting two points along the defect contour using laser tweezers. After some time, these structures relax into the eye-shape shown in Supplementary Fig. 4 . This shape is well approximated as two circular arcs of contour length l and radius r connected at points A and B and centred at points O and O ′, respectively ( Supplementary Fig. 4 ). This shape is characterized by its length d and the junction angle φ = ( DAC ), where the line ( AC ) is the tangent line to the upper arc at point A . A simple free energy model of a π -wall contains two terms. The first is the line tension per unit length γ . The second is the bending energy per unit length κ / r 2 , where r is the local radius of curvature. The equilibrium shape and size of the structure is determined by the interplay between the π -wall line tension and bending rigidity. At the junctions A and B, the net force must be zero: γ =2( γ + κ / r 2 )cos φ . Based on geometry arguments, we can write all the relevant parameters in terms of r : s = L − d , d =2 r sin φ , and l = rπφ . Therefore, the total free energy of the system between points E and B depends only on three parameters, and is given by F ( r , γ , κ )= sγ +2 l ( γ + κ / r 2 ). Using values of γ =425 k B T μm −1 and κ =200 k B T μm measured through the fluctuation spectrum, we minimize F with respect to r and find that it displays a single minimum at the equilibrium radius r *=1.0 μm at T =22 °C, and therefore d =1.9 μm and φ =69°. These estimations compare well to the experimental results of d =3.0±0.5 μm and φ =60±5°. How to cite this article : Zakhary, M. J. et al . Imprintable membranes from incomplete chiral coalescence. Nat. Commun. 5:3063 doi: 10.1038/ncomms4063 (2014).